Targeted suppression of claudin-5 decreases cerebral oedema and improves cognitive outcome following traumatic brain injury Traumatic brain injury is the leading cause of death in children and young adults globally. Malignant cerebral oedema has a major role in the pathophysiology that evolves after severe traumatic brain injury. Added to this is the significant morbidity and mortality from cerebral oedema associated with acute stroke, hypoxic ischemic coma, neurological cancers and brain infection. Therapeutic strategies to prevent cerebral oedema are limited and, if brain swelling persists, the risks of permanent brain damage or mortality are greatly exacerbated. Here we show that a temporary and size-selective modulation of the blood-brain barrier allows enhanced movement of water from the brain to the blood and significantly impacts on brain swelling. We also show cognitive improvement in mice with focal cerebral oedema following administration in these animals of short interfering RNA directed against claudin-5. These observations may have profound consequences for early intervention in cases of traumatic brain injury, or indeed any neurological condition where cerebral oedema is the hallmark pathology. Traumatic brain injury (TBI) accounts for ~20% of deaths in people 5–35-years old, accounting for 1% of all adult mortality worldwide each year [1] . In Europe alone, brain injuries cause over 66,000 deaths per annum while almost 1.6 million people are admitted to Hospital each year [2] . Indeed, more people suffer a TBI each year than the numbers diagnosed with breast, lung, prostate, brain and colon cancer combined [3] . Added to this are a range of other acute neurological injuries including acute stroke especially in the younger patient, hypoxic ischemic coma, neurological cancers, both primary and secondary metastatic disease, and brain infection [4] . Although improved diagnostic and monitoring methods, such as magnetic resonance imaging (MRI) and intracranial pressure (ICP) transducers, have been introduced, there has been little change in mortality or the treatment of acute brain swelling over the past 80 years. One of the key mediators of morbidity and mortality in cases of cerebral oedema is the associated increases in ICP due to a dramatic shift in water diffusion across the blood-brain barrier (BBB). This build up of water within the confines of the brain and its calvarium will exert dangerous increases in ICP leading to increased risks of secondary complications ( Fig. 1a,b ) [5] . 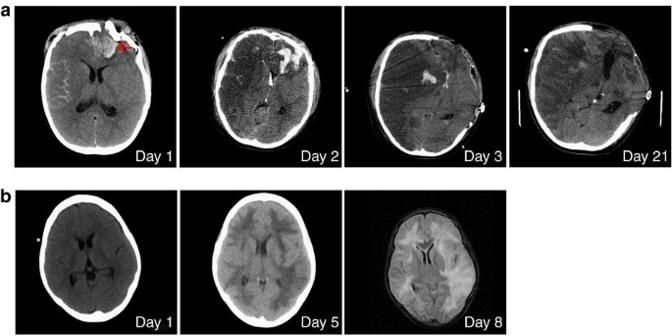Figure 1: Analysis of human cerebral oedema progression. (a) Serial axial computerized tomography (CT) scans are shown of a 12-year-old boy who suffered a severe TBI while riding an all terrain vehicle. Initial CT shows bilateral injury with a left frontal open depressed skull fracture and underlying haematoma (arrow) and right-sided subarachnoid haemorrhage (Day 1). The follow-up scan 24 h later (Day 2) shows progressive cerebral oedema due to the initial hypoxia and subsequent malignant ICPs resulting in increased right to left brain shift. The patient underwent a left-sided decompressive craniectomy (Day 3) due to refractory ICPs and the follow-up scan 3 weeks later (Day 21) shows persistent oedema despite maximal medical therapy. (b) Three images of a female patient aged 18 years admitted post-cardiac arrest. Day 1: CT scan (axial view) of the brain less than 24 h after arrest: brain parenchyma appears normal. Day 5: CT scan (axial view), showing massive generalized cerebral oedema as a result of hypoxic ischemic injury. Day 8: MRI of the brain. (T2 weighted fluid attenuated inversion recovery sequence, axial view) showing residual bilateral white matter oedema. Figure 1: Analysis of human cerebral oedema progression. ( a ) Serial axial computerized tomography (CT) scans are shown of a 12-year-old boy who suffered a severe TBI while riding an all terrain vehicle. Initial CT shows bilateral injury with a left frontal open depressed skull fracture and underlying haematoma (arrow) and right-sided subarachnoid haemorrhage (Day 1). The follow-up scan 24 h later (Day 2) shows progressive cerebral oedema due to the initial hypoxia and subsequent malignant ICPs resulting in increased right to left brain shift. The patient underwent a left-sided decompressive craniectomy (Day 3) due to refractory ICPs and the follow-up scan 3 weeks later (Day 21) shows persistent oedema despite maximal medical therapy. ( b ) Three images of a female patient aged 18 years admitted post-cardiac arrest. Day 1: CT scan (axial view) of the brain less than 24 h after arrest: brain parenchyma appears normal. Day 5: CT scan (axial view), showing massive generalized cerebral oedema as a result of hypoxic ischemic injury. Day 8: MRI of the brain. (T2 weighted fluid attenuated inversion recovery sequence, axial view) showing residual bilateral white matter oedema. Full size image The osmotic diuretic mannitol is commonly used in the acute stages of treatment of cerebral oedema, as it can establish an osmotic gradient between plasma and brain cells, reducing cerebral oedema by drawing water across areas of intact BBB into the vascular compartment [5] . Intra-arterial mannitol can also be used to enhance drug delivery to the brain in patients with brain tumours, where it is suggested it shrinks brain microvascular endothelial cells, disrupts the tight junctions at the BBB and allows chemotherapeutic drugs to access the neural environment [6] . Along with hypertonic saline, external ventricular drainage and decompressive craniectomies, it is one of the only therapeutic interventions available for cerebral oedema, with previous studies on hypothermia and steroids having demonstrated no therapeutic benefit [7] , [8] . Repeated administration of mannitol is also highly problematic as it may produce abnormal neurological and renal side effects [9] . Moreover, its effects are only beneficial for short periods and, if brain swelling continues beyond 24 h, the risks of mortality increase significantly. There are also data in children to suggest that there is a biphasic increase in malignant cerebral oedema beyond the initial 24–28 h period ( Fig. 1a ) [10] . It is now widely accepted that cerebral oedema associated with TBI involves a primary and severe disruption of the BBB at the site of injury due to endothelial cell damage, disruption of tight junction function between the endothelial cells and an induction of abnormal transcellular transport. These combined effects culminate in allowing blood-borne components to enter the brain. Indeed the resultant oedema that is formed in some cases of cerebral injury can be classified as 'vasogenic', that is, of vascular origin as is the case in the majority of TBIs and blast injuries. Ischemic forms of cerebral oedema can be termed 'cytotoxic', that is, of cellular origin, and are common in cases of acute stroke and other ischemic insults, such as cardiac arrest resulting in hypoxic ischemic coma, but in the majority of severe cases, secondary to this cytotoxic oedema, will be the vasogenic insult [11] . Although BBB dysfunction is a common hallmark of cerebral oedema, it is not well understood, and dynamic changes seem to occur in the endothelium at various time points post-injury. Initial BBB opening in diffuse closed head injury is rapid and transient, beginning immediately after impact and closing within 30 min after impact [12] . However, there seems to be a size-selectivity issue at the BBB at sites of neural damage, during the early stages post-injury, with large molecules able to diffuse into the extravascular space in the short-term and smaller molecules able to diffuse for longer periods of time [13] . This has also been shown in cases of cytotoxic injury associated with the middle cerebral artery occlusion animal model of experimental stroke [14] . It is clear that a fluctuation in the transcriptional and post-translational control of tight junction protein expression is associated with the pathology of oedema. Using RNA interference targeting the tight junction component claudin-5, we show that the BBB can be modulated to enhance the exchange of very low molecular weight molecules of up to ~1 kDa for periods of between 24 and 72 h post-injection, with no apparent negative phenotypic or genotypic effects on experimental animals [15] , [16] , [17] . Claudin-5 has a key role in the formation of paracellular pores or channels that function in mediating selective ion permeability at the BBB [18] , [19] . It has previously been reported that dynamic changes occur at the level of tight junction protein expression at the BBB in response to TBI, with levels of claudin-5, occludin and ZO-1 being transcriptionally regulated at various time points post-injury [20] . While these changes have traditionally been purported to represent a pathological hallmark of oedema, we suggest that the initial decreases in tight junction protein expression are in direct response to fluid accumulation in the extra-cellular micro-environment. We hypothesized that size-selective modulation of the BBB allows for enhanced paracellular diffusion of extra-neural water accumulated as a result of vasogenic oedema ( Supplementary Fig. S1 ) and, to this end, we administered short interfering (siRNA) directed against claudin-5 post induction of a focal cerebral oedema, finding that this attenuated the oedema and its comorbidities. Efficacy of systemic administration of claudin-5 siRNA Claudin-5 siRNA was assessed for efficacy in mouse b.End3 brain microvascular endothelial cells, and an optimum sequence was selected for in vivo studies ( Fig. 2a,b ). For in vivo use, claudin-5 siRNA was complexed with the cationic polymer in vivo-jetPEI and formed stable particles with a zeta potential of ~37 mV, which is an indication of a stable particle with gross positive charge and will allow for ease of diffusion into endothelial cells ( Fig. 2c ). Conjugated siRNA-Cy3/ in vivo-jetPEI complexes were injected into the mouse tail vein to assess bio-distribution and showed efficient transfection of the brain, liver and lung microvascular endothelium, with siRNA persisting in tissues for between 24 h and 48 h post-injection ( Fig. 2d ). It is important to note that claudin-5 is more highly enriched in the brain than any other organ including the lung, liver, or heart [21] . Preparation of capillary-isolated brain fractions, 48 h after systemic administration of claudin-5 siRNA, showed efficient suppression of claudin-5 levels, which has previously been shown to be reversible [15] ( Fig. 2e ). This suppression was manifested by decreased levels of claudin-5 at the endothelial cell peripheries ( Fig. 2f ) and MRI analysis (using Gd-DTPA contrast agent) showed distinct differences between mice receiving a non-targeting control (NT) siRNA and mice receiving claudin-5 siRNA ( Fig. 2g ). Bolus chase analysis showed an initial decrease in the T1 longitudinal relaxation rate and a slower rate of recovery to the baseline signal, indicating the persistence of the contrast agent in some regions of the cortical neural tissue and providing a direct correlation that the BBB was modulated ( Fig. 2h ). Importantly, there were no significant abnormalities detected following histopathological analysis of major organs in mice receiving either NT siRNA or claudin-5 siRNA when compared with un-injected mice ( Supplementary Fig. S2 ). Moreover, blood biochemistry analysis of mice post-injection with NT siRNA or claudin-5 siRNA did not reveal any overt differences compared with un-injected mice ( Supplementary Table S1 ). There were single base changes in the target mRNA sequence between rodents, humans and non-human primates ( Supplementary Table S2 ). 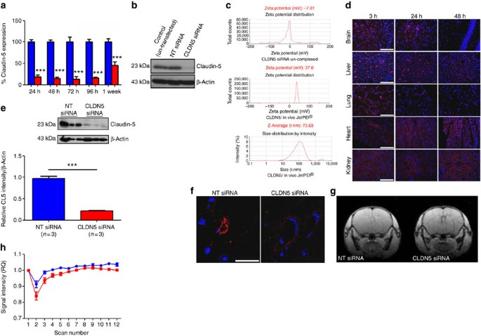Figure 2: Suppression efficacy of mouse claudin-5 siRNA and phenotype analysis. (a) Claudin-5 levels were significantly (***P≤0.0001, ANOVA with Tukey's post test) decreased in mouse bEnd.3 endothelial cell line at the transcript level, blue bars (NT siRNA,n=3), red bars (CLDN5 siRNA,n=3), data are means±s.e.m. and (b) at the protein level. (c) Un-complexed siRNA gave a negative zeta-potential reading of −7.81 mV (top panel), when complexed within vivo-jetPEIsolution, the zeta-potential was increased to 37 mV (middle panel) and formed particles with a size of ~73.63 nm (bottom panel). (d) siRNA conjugated to the fluorescent dye Cy3 (siRNA-Cy3: red, DAPI: blue) efficiently transfected brain microvascular endothelial cells (top row) and persisted for up to 24 h post-injection. siRNA persisted in the liver (second row) up to 24 h with low levels still apparent 48 h post-injection. Levels of siRNA were only evident in the lung (third row) up to 24 h post-injection with very little levels detected at 48 h. Minimal siRNA was detected in the heart or kidney (fourth and fifth rows), scale bars, ~100 μm. (e) Levels of claudin-5 were significantly (***P≤0.0001, Studentst-test,n=3 per group, data are means±s.e.m.) decreased in capillary fractions of mouse brains 48 h post-injection of siRNA/in vivo-jetPEIcomplexes. (f) Immunohistochemical analysis showed a discontinuous pattern of claudin-5 staining post-injection of claudin-5 siRNA. Scale bar, 100 μm. (g) T-1 weighted contrast enhanced MR images showed distinctive extravasation of Gd-DTPA (742 Da) 48 h post-injection of claudin-5 siRNA compared with NT siRNA. (h) Following tail vein injection of Gd-DTPA, bolus chase analysis of the contrast agent in a cortical region of the mouse brain showed a slower clearance rate of Gd-DTPA in the claudin-5 siRNA (red line,n=8) group compared with the NT siRNA group (blue line,n=6). Figure 2: Suppression efficacy of mouse claudin-5 siRNA and phenotype analysis. ( a ) Claudin-5 levels were significantly (*** P ≤0.0001, ANOVA with Tukey's post test) decreased in mouse bEnd.3 endothelial cell line at the transcript level, blue bars (NT siRNA, n =3), red bars (CLDN5 siRNA, n =3), data are means±s.e.m. and ( b ) at the protein level. ( c ) Un-complexed siRNA gave a negative zeta-potential reading of −7.81 mV (top panel), when complexed with in vivo-jetPEI solution, the zeta-potential was increased to 37 mV (middle panel) and formed particles with a size of ~73.63 nm (bottom panel). ( d ) siRNA conjugated to the fluorescent dye Cy3 (siRNA-Cy3: red, DAPI: blue) efficiently transfected brain microvascular endothelial cells (top row) and persisted for up to 24 h post-injection. siRNA persisted in the liver (second row) up to 24 h with low levels still apparent 48 h post-injection. Levels of siRNA were only evident in the lung (third row) up to 24 h post-injection with very little levels detected at 48 h. Minimal siRNA was detected in the heart or kidney (fourth and fifth rows), scale bars, ~100 μm. ( e ) Levels of claudin-5 were significantly (*** P ≤0.0001, Students t -test, n =3 per group, data are means±s.e.m.) decreased in capillary fractions of mouse brains 48 h post-injection of siRNA/ in vivo-jetPEI complexes. ( f ) Immunohistochemical analysis showed a discontinuous pattern of claudin-5 staining post-injection of claudin-5 siRNA. Scale bar, 100 μm. ( g ) T-1 weighted contrast enhanced MR images showed distinctive extravasation of Gd-DTPA (742 Da) 48 h post-injection of claudin-5 siRNA compared with NT siRNA. ( h ) Following tail vein injection of Gd-DTPA, bolus chase analysis of the contrast agent in a cortical region of the mouse brain showed a slower clearance rate of Gd-DTPA in the claudin-5 siRNA (red line, n =8) group compared with the NT siRNA group (blue line, n =6). Full size image Claudin-5 siRNA alters the BBB dysfunction phenotype Cold-induced cerebral oedema produces an injury that results in the development of focally extensive well-demarcated regions of necrosis typically within the grey matter of the visual and somatosensory cortex of the right cerebral hemisphere ( Fig. 3a ). Brain parenchymal necrosis was characterized by the formation of a well-demarcated solid coagulums of denatured parenchymal proteins. Within these foci, some blood vessels were spared or had proliferated (an angiogenic response). At the periphery of these foci, there was gliosis, characterized by a prominence of astrocytes, microglia, neutrophils and occasional lymphocytes ( Fig. 3b ). Multifocal haemorrhages occured within the necrotic area and at the margins, with blood vessel endothelia in these areas typically showing signs of activation with large plump endothelial cells with nuclei containing prominent nucleoli ( Fig. 3c ). 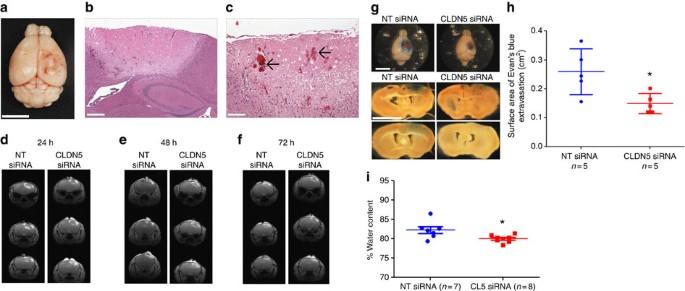Figure 3: Cold-induced cerebral oedema and the effect of barrier modulation in a brain injury model. (a) Cold-induced cerebral injury created a focal vasogenic oedema in the right hemisphere of the mouse brain. Scale bar, 5 mm. (b) The focal injury extended as far as the hippocampus and created a large region of focal necrosis. Scale bar, 250 μm. (c) Neutrophil extravasation and endothelial cell activation are apparent along with haemmorrage (arrows). Scale bar, 100 μm. (d) Contrast-enhanced MRI shows the TBI region post-Gd-DTPA infusion in NT siRNA-injected mice (left panels) and claudin-5 siRNA-injected mice (right panels) 24 h post-injury. (e) NT siRNA-injected mice (left panel) and claudin-5 siRNA-injected mice (right panel) 48 h post-injury and (f) NT siRNA-injected mice (left panel) and claudin-5 siRNA-injected mice (right panel) 72 h post-injury. (g) Surface, cortical extravasation of Evan's blue (blue staining) was observed in NT siRNA-injected mice and claudin-5 siRNA-injected mice 48 h post-injury (left and right panels respectively; scale bar, 5 mm). Cross-sections of the injured areas were observed in both experimental groups in the panels below. Scale bars 5 mm. (h) Quantification of the surface area of Evan's blue extravastaion was assessed in both experimental groups (*P=0.0464, Student'st-test,n=5 for each group). (i) Percentage water content as calculated by wet/dry weights was significantly decreased at the site of injury in claudin-5 siRNA-injected mice (*P=0.0224, Student'st-test, NT siRNAn=7, claudin-5 siRNAn=8). Figure 3: Cold-induced cerebral oedema and the effect of barrier modulation in a brain injury model. ( a ) Cold-induced cerebral injury created a focal vasogenic oedema in the right hemisphere of the mouse brain. Scale bar, 5 mm. ( b ) The focal injury extended as far as the hippocampus and created a large region of focal necrosis. Scale bar, 250 μm. ( c ) Neutrophil extravasation and endothelial cell activation are apparent along with haemmorrage (arrows). Scale bar, 100 μm. ( d ) Contrast-enhanced MRI shows the TBI region post-Gd-DTPA infusion in NT siRNA-injected mice (left panels) and claudin-5 siRNA-injected mice (right panels) 24 h post-injury. ( e ) NT siRNA-injected mice (left panel) and claudin-5 siRNA-injected mice (right panel) 48 h post-injury and ( f ) NT siRNA-injected mice (left panel) and claudin-5 siRNA-injected mice (right panel) 72 h post-injury. ( g ) Surface, cortical extravasation of Evan's blue (blue staining) was observed in NT siRNA-injected mice and claudin-5 siRNA-injected mice 48 h post-injury (left and right panels respectively; scale bar, 5 mm). Cross-sections of the injured areas were observed in both experimental groups in the panels below. Scale bars 5 mm. ( h ) Quantification of the surface area of Evan's blue extravastaion was assessed in both experimental groups (* P =0.0464, Student's t -test, n =5 for each group). ( i ) Percentage water content as calculated by wet/dry weights was significantly decreased at the site of injury in claudin-5 siRNA-injected mice (* P =0.0224, Student's t -test, NT siRNA n =7, claudin-5 siRNA n =8). Full size image The injured region of the brain displayed a 'biphasic' opening of the BBB at the penumbral region sub-adjacent to the injury site. This BBB opening was evident 24 h post-injury ( Fig. 3d ) but was not apparent 48 h ( Fig. 3e ) after the injury in the NT siRNA-injected mice. Interestingly, the opening in the penumbra returned 72 h ( Fig. 3f ) after the injury albeit with less intensity in NT siRNA-injected animals. However, in mice receiving claudin-5 siRNA, the penumbral region displayed extravasation of Gd-DTPA that persisted up to and including 72 h post-injection of siRNA ( Fig. 3d–f ). To assess the BBB phenotype at the injury site to a larger molecular weight tracer, we employed Evan's blue dye. Evan's blue is a low molecular weight dye commonly used for the evaluation of BBB dysfunction. However, it must be noted that it potently binds to circulating albumin and its extravasation is indicative of severe BBB breakdown and albumin (70 kDa MW) leakage into the parenchyma. Evan's blue dye was injected in mice 24 h post-injury in animals receiving either NT siRNA or claudin-5 siRNA. We observed a significant decrease in the amount of Evan's blue extravasation at the site of injury in mice that received the claudin-5 siRNA complexes ( Fig. 3g ) as manifested by the surface 'spread' of dye leakage in the cortical region of the injury. Cross-section analysis of the brains at the injured regions showed that Evan's blue extravasation was less evident in the claudin-5 siRNA-injected mice ( Fig. 3g ) and this observation was significant (* P ≤0.05) ( Fig. 3h , histogram). Percentage water content in the injured brain region of mice, receiving claudin-5 siRNA, was also significantly decreased compared with the injured brain regions of mice receiving NT siRNA ( Fig. 3i ). Barrier modulation decreases lesion volume To assess whether BBB modulation could impact on the development of lesion size at the site of injury, mice were analysed using high-resolution T-2 weighted MRI 24, 48 and 72 h post-siRNA-injection. There was a significant decrease in lesion volume 72 h post-injury in mice receiving claudin-5 siRNA (* P =0.0344) ( Fig. 4a ). This was manifested as an overall decrease in the injured region in the colour-enhanced three-dimensional rendered images ( Supplementary Fig. S3 ) and in each orientation of the injury site analysed ( Fig. 4b ). Indeed, siRNAs injected 6 h and 24 h post-TBI also elicited significant decreases in TBI volume, a result that holds strong clinical relevance ( Fig. 5 ). We also observed that the lower limit of efficacy for claudin-5 siRNA was 10 μg, as no significant differences in lesion volumes were observed at this dose ( Supplementary Fig. S4 ). 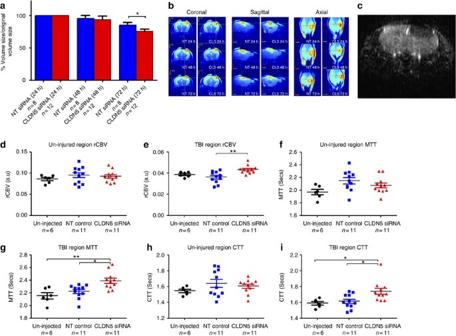Figure 4: Claudin-5 siRNA decreases lesion volume and cerebral oedema formation. (a) Volumetric analysis of lesion volume post-TBI showed a significant decrease from baseline 72 h post-injection of claudin-5 siRNA (*P≤0.05, Student'st-test, NT siRNA,n=8, CLDN5 siRNA,n=12. Data are means±s.e.m.). (b) Orientation of pseudo-coloured high-resolution MR images showed mice in the coronal, sagittal and axial planes at the site of injury and at each time point post-injury, NT siRNA-injected mice are in the left panel of each orientation whereas claudin-5 siRNA-injected mice are in the right panel. (c) Region of interest analysed in ASL measurements. (d) No significant difference in relative cerebral blood flow (rCBV) in control ROI between groups. (e) rCBV is significantly higher in claudin-5 siRNA-injected mice than in NT siRNA-injected mice (**P<0.01) (One way ANOVA, Bonferroni post test for multiple comparisons, 95% confidence interval). (f) No significant difference in MTT in control ROI between groups. (g) MTT is significantly higher in claudin-5 siRNA-injected mice than in control (**P<0.01) and NT siRNA-injected mice (*P<0.05), (One-way ANOVA, Bonferroni post test for multiple comparisons, 95% confidence interval). (h) No significant difference in CTT in control ROI between groups. (i) CTT is significantly higher in claudin-5 siRNA-injected mice than in control (*P<0.05) and NT siRNA-injected mice (*P<0.05), (One-way ANOVA, Bonferroni post test for multiple comparisons, 95% confidence interval). Figure 4: Claudin-5 siRNA decreases lesion volume and cerebral oedema formation. ( a ) Volumetric analysis of lesion volume post-TBI showed a significant decrease from baseline 72 h post-injection of claudin-5 siRNA (* P ≤0.05, Student's t -test, NT siRNA, n =8, CLDN5 siRNA, n =12. Data are means±s.e.m.). ( b ) Orientation of pseudo-coloured high-resolution MR images showed mice in the coronal, sagittal and axial planes at the site of injury and at each time point post-injury, NT siRNA-injected mice are in the left panel of each orientation whereas claudin-5 siRNA-injected mice are in the right panel. ( c ) Region of interest analysed in ASL measurements. ( d ) No significant difference in relative cerebral blood flow (rCBV) in control ROI between groups. ( e ) rCBV is significantly higher in claudin-5 siRNA-injected mice than in NT siRNA-injected mice (** P <0.01) (One way ANOVA, Bonferroni post test for multiple comparisons, 95% confidence interval). ( f ) No significant difference in MTT in control ROI between groups. ( g ) MTT is significantly higher in claudin-5 siRNA-injected mice than in control (** P <0.01) and NT siRNA-injected mice (* P <0.05), (One-way ANOVA, Bonferroni post test for multiple comparisons, 95% confidence interval). ( h ) No significant difference in CTT in control ROI between groups. ( i ) CTT is significantly higher in claudin-5 siRNA-injected mice than in control (* P <0.05) and NT siRNA-injected mice (* P <0.05), (One-way ANOVA, Bonferroni post test for multiple comparisons, 95% confidence interval). 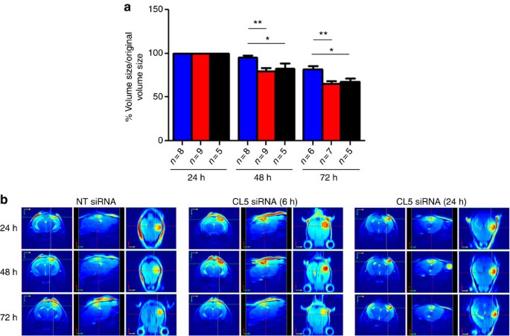Figure 5: Analysis of lesion volumes when siRNA is administered 6 and 24 h post-injury. (a) Claudin-5 siRNA was administered 6 h (red bars) or 24 h (black bars) post-injury, and compared to NT siRNA-administered animals (blue bars). Significant decreases in lesion volume were observed 48 h (**P≤0.01 and *P≤0.05 for 6 h and 24 h injections, respectively, ANOVA with Tukey's post test, NT siRNAn=8, claudin-5 siRNA 6 hn=9, claudin-5 siRNA 24 hn=5) and 72 h post-injection of claudin-5 siRNA (**P≤0.01 and *P≤0.05 for 6 h and 24 h injections, respectively, ANOVA with Tukey's post test, NT siRNAn=6, claudin-5 siRNA 6 hn=7, claudin-5 siRNA 24 hn=5) at both time points compared with NT siRNA-injected mice (blue bars). Data are means±s.e.m. (b) Representatives of coronal (left columns), sagittal (middle columns) and axial (right columns) planes at the site of injury. Full size image Figure 5: Analysis of lesion volumes when siRNA is administered 6 and 24 h post-injury. ( a ) Claudin-5 siRNA was administered 6 h (red bars) or 24 h (black bars) post-injury, and compared to NT siRNA-administered animals (blue bars). Significant decreases in lesion volume were observed 48 h (** P ≤0.01 and * P ≤0.05 for 6 h and 24 h injections, respectively, ANOVA with Tukey's post test, NT siRNA n =8, claudin-5 siRNA 6 h n =9, claudin-5 siRNA 24 h n =5) and 72 h post-injection of claudin-5 siRNA (** P ≤0.01 and * P ≤0.05 for 6 h and 24 h injections, respectively, ANOVA with Tukey's post test, NT siRNA n =6, claudin-5 siRNA 6 h n =7, claudin-5 siRNA 24 h n =5) at both time points compared with NT siRNA-injected mice (blue bars). Data are means±s.e.m. ( b ) Representatives of coronal (left columns), sagittal (middle columns) and axial (right columns) planes at the site of injury. Full size image Using arterial spin labelling (ASL) (a non-invasive MRI technique that uses magnetically labelled arterial blood water in the neck as an endogenous tracer to characterize cerebral perfusion) [22] , perfusion-weighted images were generated. Experimental data were fitted to a recently developed quantitative model of cerebral perfusion to quantify mean transit time (MTT), capillary transit time (CTT) and relative cerebral blood volume (rCBV) [23] , [24] . The MTT represents the time taken for labelled water to travel from the labelling plane in the neck to the imaging plane in the brain. The CTT is a measure of the dispersion of labelled water at the imaging plane due to exchange of water from the vasculature to the brain tissue and pseudo-diffusion within the microvessels. rCBV was obtained from the amplitude of the ASL signal in the selected region of interest (ROI) as outlined in Fig. 4c . No significant differences in rCBV in the contralateral control un-injured brain region were identified in any experimental group ( Fig. 4d ). However, it is worth noting the large difference in rCBV in the control ROI versus the TBI ROI ( Fig. 4e ). Importantly, mice injected with claudin-5 siRNA had a significant increase in rCBV that trended towards the control (contralateral to TBI ROI), un-injured rCBV (** P ≤0.01) ( Fig. 4e ). This observation suggests a recovery of rCBV in the injured ROI of mice receiving claudin-5 siRNA. Concomitantly, when we assessed the MTT in the injured ROI of the claudin-5 siRNA-injected group, we observed a significantly higher MTT than in the other two groups (* P ≤0.05) ( Fig. 4g ). MTT is a measurement of blood volume over blood flow. When combined with the measured increase in rCBV above, we hypothesize that this increase in MTT is most likely due to an increase in blood volume in the injured ROI rather than a decrease in blood flow ( Fig. 4f ). To assess the rates of exchange of water in the tissue, CTT was also assessed and was observed to be significantly higher in the injured ROI of mice receiving claudin-5 siRNA than in the other two groups (* P ≤0.05) ( Fig. 4i ). CTT is a measurement of perfusion coefficient/flow 2 , and our findings imply that the perfusion coefficient, P , has increased (where P , having units of diffusion, represents dispersion of the magnetically labelled water at the ROI due to pseudo diffusion within the microvasculature and the exchange of labelled water from the capillary bed to the tissue and vice versa). CTT values did not differ in the un-injured ROI of any experimental groups ( Fig. 4h ). Overall, at the site of the injury, the ASL results suggested much less exchange from capillaries into tissue but a significant recovery was observed in the claudin-5 siRNA-injected animals. Cytokine profile and dynamic of injured neuronal tissue TBI-induced neuroinflammatory changes have long been cited as being central to oedema progression [25] , yet the role of inflammatory cytokines and their impact on oedema formation is less clear. Therefore, following injury and injection with NT or claudin-5 siRNA, we analysed the transcriptional profile of a range of neuroinflammatory-associated cytokines 24 and 48 h post-injury. We also undertook a series of cytokine proteome arrays to elucidate distinct changes between experimental groups. Transcriptional analysis of these neuroinflammatory markers showed marked differences between mice injected with NT siRNA compared with those receiving claudin-5 siRNA. In particular, transcript levels of C-X-C motif chemokine 10 (CXCL10) and for Interleukin-1Beta (IL-1β) were significantly increased in claudin-5 siRNA compared with NT siRNA-injected mice 24 h post-injury ( Fig. 6a,b ). Levels of cytokine-induced neutrophil chemoattractant-1 (Cinc-1), transforming growth factor (TGF), tumour necrosis factor alpha (TNF-α), glial-derived neurotrophic factor (GDNF), and nerve growth factor (NGF) were differentially regulated at various times post-treatment with claudin-5 siRNA ( Fig. 6c–g ). No significant differences were observed in levels of interleukin-10 (IL-10), inter-cellular adhesion molecule-1 (ICAM-1), regulated on activation, normal T-cell expressed and secreted (RANTES), brain-derived neurotrophic factor (BDNF) and vascular cell adhesion molecule-1 (VCAM-1) ( Supplementary Fig. S5 ). 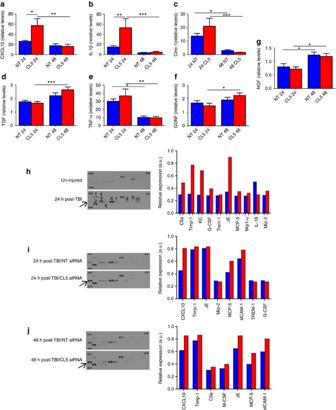Figure 6: Cytokine profiling of injured brain region post-injection of siRNA. (a) CXCL10 transcript levels were increased in the injured region of claudin-5 siRNA-injected mice compared with NT siRNA-injected mice 24 h post-injury (*P≤0.05, NTn=8, claudin-5n=8). These levels decreased in claudin-5 siRNA-injected mice from 24 to 48 h (**P≤0.01, 24 hn=8, 48 hn=8). (b) IL-1β levels were increased in claudin-5 siRNA-injected mice compared with NT siRNA-injected mice at 24 h (**P≤ 0.01, NTn=8, claudin-5n=6). These levels decreased at 48 h (***P≤0.001, NT 24 hn=, 48 hn=7, claudin-5 24 hn=6, 48 hn=8). (c) Cinc-1 levels decreased in both groups (NT siRNA and claudin-5 siRNA) from 24 to 48 h (***P≤0.001, NT 24 hn=7, 48 hn=7, claudin-5 24 hn=6, 48 hn=7). (d) TGF-β levels increased in claudin-5 siRNA-injected mice from 24 to 48 h (***P≤0.001, 24 hn=8, 48 hn=8). (e) TNF-α levels decreased in both groups from 48 to 24 h (*P≤0.05, **P≤0.01, respectively, NT 24 hn=8, 48 hn=7, claudin-5 24 hn=8, 48 hn=8). (f) GDNF levels increased in claudin-5 siRNA-injected mice from 24 to 48 h (*P≤0.05, 24 hn=8, 48 hn=8). (g) NGF levels increased in both groups from 24 to 48 h (*P≤0.05, NT 24 hn=8, 48 hn=7, claudin-5 24 hn=8, 48 hn=7). All data are ANOVA with Tukey's post-test, illustrated as mean±s.e.m. (h) Cytokine proteome array profiling identified the following proteins upregulated at the injury site, 1: C5a, 2: Timp-1 3: KC, 4: G-CSF, 5: Trem-1, 6: JE, 7: MCP-5, 8: Mip1-α, 9: IL-16, 10: Mip-2. Blue=uninjured, red=injured. (i) CXCL10 (arrow) was increased 60% in the region 24 h post-claudin-5 siRNA compared with NT siRNA. Levels of MCP-5 and sICAM-1 were also increased by ~30%. Blue=NT, red=claudin-5. (j) JE was higher in claudin-5 siRNA-injected mice by ~20% at 48 h. CXCL10, MCP-5 and sICAM-1 remained higher at 48 h. Figure 6: Cytokine profiling of injured brain region post-injection of siRNA. ( a ) CXCL10 transcript levels were increased in the injured region of claudin-5 siRNA-injected mice compared with NT siRNA-injected mice 24 h post-injury (* P ≤0.05, NT n =8, claudin-5 n =8). These levels decreased in claudin-5 siRNA-injected mice from 24 to 48 h (** P ≤0.01, 24 h n =8, 48 h n =8). ( b ) IL-1β levels were increased in claudin-5 siRNA-injected mice compared with NT siRNA-injected mice at 24 h (** P ≤ 0.01, NT n =8, claudin-5 n =6). These levels decreased at 48 h (*** P ≤0.001, NT 24 h n =, 48 h n =7, claudin-5 24 h n =6, 48 h n =8). ( c ) Cinc-1 levels decreased in both groups (NT siRNA and claudin-5 siRNA) from 24 to 48 h (*** P ≤0.001, NT 24 h n =7, 48 h n =7, claudin-5 24 h n =6, 48 h n =7). ( d ) TGF-β levels increased in claudin-5 siRNA-injected mice from 24 to 48 h (*** P ≤0.001, 24 h n =8, 48 h n =8). ( e ) TNF-α levels decreased in both groups from 48 to 24 h (* P ≤0.05, ** P ≤0.01, respectively, NT 24 h n =8, 48 h n =7, claudin-5 24 h n =8, 48 h n =8). ( f ) GDNF levels increased in claudin-5 siRNA-injected mice from 24 to 48 h (* P ≤0.05, 24 h n =8, 48 h n =8). ( g ) NGF levels increased in both groups from 24 to 48 h (* P ≤0.05, NT 24 h n =8, 48 h n =7, claudin-5 24 h n =8, 48 h n =7). All data are ANOVA with Tukey's post-test, illustrated as mean±s.e.m. ( h ) Cytokine proteome array profiling identified the following proteins upregulated at the injury site, 1: C5a, 2: Timp-1 3: KC, 4: G-CSF, 5: Trem-1, 6: JE, 7: MCP-5, 8: Mip1-α, 9: IL-16, 10: Mip-2. Blue=uninjured, red=injured. ( i ) CXCL10 (arrow) was increased 60% in the region 24 h post-claudin-5 siRNA compared with NT siRNA. Levels of MCP-5 and sICAM-1 were also increased by ~30%. Blue=NT, red=claudin-5. ( j ) JE was higher in claudin-5 siRNA-injected mice by ~20% at 48 h. CXCL10, MCP-5 and sICAM-1 remained higher at 48 h. Full size image We also used a mouse cytokine proteome array to elucidate the protein levels of cytokines in the injured brain region. Initially, a direct comparison of un-injured and injured cortical tissue showed a range of cytokines upregulated in the injured tissue. Interestingly there was a decrease in interleukin-16 (IL-16) expression at the injury site compared with the un-injured tissue samples ( Fig. 6h ). Furthermore, we observed a range of differentially expressed proteins between the 2 experimental cohorts, 24 h and 48 h post-injury, with a 60% increase in CXCL10 levels in the claudin-5 siRNA-injected animals compared with the NT siRNA-injected mice that persisted up to and including 48 h post-injury ( Fig. 6i,j ), reflecting our observations at the transcript level. Levels of other cytokines including MCP-5 and sICAM-1 were also increased in mice receiving claudin-5 siRNA compared with those receiving NT siRNA 24 h and 48 h post-injury ( Fig. 6i,j ). Given the extensive data available that siRNAs can induce toll-like receptor (TLR)-mediated inflammatory responses in cells in vitro and in vivo [26] , we wished to determine the inflammatory profile of claudin-5 siRNA compared with both NT siRNA and a 2′OMe-modified claudin-5 siRNA. It has been shown that 2′OMe backbone modifications in even 2 residues of an siRNA can abrogate these effects and, in this regard, we designed an siRNA with 2 modifications in the sense strand of the siRNA [27] . We complexed this siRNA with in vivo-jetPEI and injected the complexes into the tail veins of mice. We observed strong suppression of claudin-5 in the capillary isolations prepared from the brain samples 48 h post-injection ( Fig. 7a ). Moreover, we isolated bone-marrow derived macrophages (BMDMs) from WT C57/Bl6 mice. Cells were treated with siRNA for 24 h, and transcript levels of interferon-α were subsequently analysed and shown to be significantly increased in NT siRNA-treated cells compared with untreated cells and claudin-5 siRNA and 2′OMe-modified siRNA-treated cells ( Fig. 7b ). All of these changes were decreased when siRNAs were complexed with in vivo-jetPEI . We also isolated peripheral myeloid from the bloods of mice 24 h post-injection of siRNAs and found no interferon-α expression when compared with positive controls (known ligands for TLR7, TLR3 and TLR4) ( Fig. 7c ). 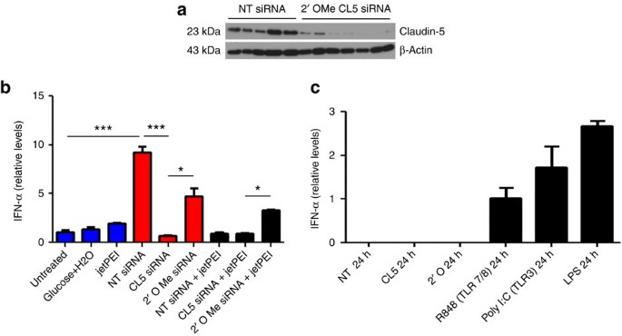Figure 7: Analysis of suppression efficacy of 2′OMe-modified claudin-5 siRNA and interferon-α expression. (a) 2′OMe-modified claudin-5 siRNA was designed with 2 modifications in the sense strand. Modified claudin-5 siRNA caused suppression of claudin-5 in brain capillary isolates. (b) In BMDMs treated with NT siRNA, a significant upregulation of interferon-α was observed compared with untreated, glucose-treated orin vivo-jetPEI™ treated cells (***P≤0.0001, ANOVA with Tukey's post test, NT siRNA,n=4, claudin-5 siRNA,n=5). Levels were also significantly increased in NT siRNA treated cells when compared with claudin-5 siRNA (***P≤0.0001, ANOVA with Tukey's post test, NT siRNA,n=4, claudin-5 siRNA,n=5). 2′OMe-modified claudin-5 siRNA-treated cells expressed significantly higher interferon-α when compared with un-modified claudin-5 siRNA (*P≤0.05, ANOVA with Tukey's post-test, NT siRNA,n=4, claudin-5 siRNA,n=5). siRNA's complexed within vivo-jetPEIproduced an overall decreased level of interferon-α expression. (c) Tail vein administration of NT siRNA, claudin-5 siRNA or 2′OMe-modified claudin-5 siRNA showed no significant increases in interferon-α expression when compared with positive controls (poly I:C-TLR3, R848-TLR7 and LPS-TLR4). Figure 7: Analysis of suppression efficacy of 2′OMe-modified claudin-5 siRNA and interferon-α expression. ( a ) 2′OMe-modified claudin-5 siRNA was designed with 2 modifications in the sense strand. Modified claudin-5 siRNA caused suppression of claudin-5 in brain capillary isolates. ( b ) In BMDMs treated with NT siRNA, a significant upregulation of interferon-α was observed compared with untreated, glucose-treated or in vivo-jetPEI ™ treated cells (*** P ≤0.0001, ANOVA with Tukey's post test, NT siRNA, n =4, claudin-5 siRNA, n =5). Levels were also significantly increased in NT siRNA treated cells when compared with claudin-5 siRNA (*** P ≤0.0001, ANOVA with Tukey's post test, NT siRNA, n =4, claudin-5 siRNA, n =5). 2′OMe-modified claudin-5 siRNA-treated cells expressed significantly higher interferon-α when compared with un-modified claudin-5 siRNA (* P ≤0.05, ANOVA with Tukey's post-test, NT siRNA, n =4, claudin-5 siRNA, n =5). siRNA's complexed with in vivo-jetPEI produced an overall decreased level of interferon-α expression. ( c ) Tail vein administration of NT siRNA, claudin-5 siRNA or 2′OMe-modified claudin-5 siRNA showed no significant increases in interferon-α expression when compared with positive controls (poly I:C-TLR3, R848-TLR7 and LPS-TLR4). Full size image Improved cognitive function in claudin-5 siRNA-injected mice Neurological severity scoring (NSS) has previously been shown to strongly correlate with the extent of TBI in a range of animal model systems [28] . We used a 10-point NSS scale that has been described previously and has been adapted for use with our model system. NSS was used to ascertain motor and cognitive function in mice post-injury and all tests were carried out by an individual blinded to the experimental treatment. We observed significantly improved NSS scores in mice that received claudin-5 siRNA compared with NT siRNA, and this effect was manifested even as early as 8 h post-injury and persisted up to and including 1 week post-injury ( Fig. 8a ). 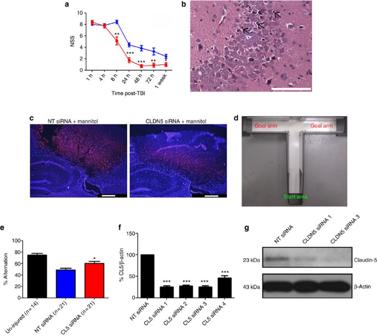Figure 8: Improvement in cognitive outcome in mice receiving claudin-5 siRNA. (a) NSS was significantly decreased in mice administered claudin-5 siRNA directly after injury. NSS benefit manifested 8 h post-injury (**P=0.0011,Student'st-test), 24 h (***P=0.0004, Student'st-test), 48 h (***P≤0.0001, Student'st-test) and 72 h (**P=0.0035, Student'st-test) in claudin-5 siRNA-injected mice and remained up to and including 1 week (*P=0.0122, Student'st-test) post-injury compared with mice receiving an injury and NT siRNA, blue line (NT siRNA,n=8), red line (CLDN5 siRNA,n=8). (b) Cold-induced injury caused necrosis as far as cells in CA1 of the hippocampus (necrotic cells indicated by arrows). Scale bar, 20 μm. (c) TUNEL (red) staining of the injured brain region from mice receiving NT siRNA or claudin-5 siRNA showed a marked decrease in the number of TUNEL-positive cells in the CA1 region of the hippocampus (DAPI: blue). Scale bars, 250 μm. Both groups of mice also received mannitol by IP injection (d) The T-maze consisted of a wooden maze with 3 arms, 2 of them situated at 180° from each other, and the third, representing the stem arm of the T, situated at 90° with respect to the other 2. All arms were 35-cm long, 6-cm wide and enclosed by 18-cm black walls. Two identical guillotine doors were placed in the entry of the goal arms and one guillotine door was situated at the end of the stem arm (start area). (e) Un-injured mice (n=14) displayed alternating behaviour with a mean alternation of 74%. Mice receiving NT siRNA (n=21) post-injury displayed decreased alternating behaviour to a mean of 48.8%, while mice receiving claudin-5 siRNA (n=21) post-injury showed a significant increase in alternating behaviour (*P≤0.05, ANOVA with Tukey's post-test) with a mean of 60.5% alternating behaviour. (f) Four individual siRNAs designed to target different regions of the human claudin-5 mRNA were designed and screened using qPCR. All siRNA's displayed efficient suppression (***P≤0.0001, ANOVA with Tukey's post-test,n=3 for each group) and claudin-5 siRNA 1 and claudin-5 siRNA 3 were chosen because of their target region homology with all major non-human primates. (g) Western blot analysis of claudin-5 levels post-transfection of claudin-5 siRNA 1 and claudin-5 siRNA 3 showed efficient suppression of claudin-5 at the protein level. Figure 8: Improvement in cognitive outcome in mice receiving claudin-5 siRNA. ( a ) NSS was significantly decreased in mice administered claudin-5 siRNA directly after injury. NSS benefit manifested 8 h post-injury (** P =0.0011,Student's t -test), 24 h (*** P =0.0004, Student's t -test), 48 h (*** P ≤0.0001, Student's t -test) and 72 h (** P =0.0035, Student's t -test) in claudin-5 siRNA-injected mice and remained up to and including 1 week (* P =0.0122, Student's t -test) post-injury compared with mice receiving an injury and NT siRNA, blue line (NT siRNA, n =8), red line (CLDN5 siRNA, n =8). ( b ) Cold-induced injury caused necrosis as far as cells in CA1 of the hippocampus (necrotic cells indicated by arrows). Scale bar, 20 μm. ( c ) TUNEL (red) staining of the injured brain region from mice receiving NT siRNA or claudin-5 siRNA showed a marked decrease in the number of TUNEL-positive cells in the CA1 region of the hippocampus (DAPI: blue). Scale bars, 250 μm. Both groups of mice also received mannitol by IP injection ( d ) The T-maze consisted of a wooden maze with 3 arms, 2 of them situated at 180° from each other, and the third, representing the stem arm of the T, situated at 90° with respect to the other 2. All arms were 35-cm long, 6-cm wide and enclosed by 18-cm black walls. Two identical guillotine doors were placed in the entry of the goal arms and one guillotine door was situated at the end of the stem arm (start area). ( e ) Un-injured mice ( n =14) displayed alternating behaviour with a mean alternation of 74%. Mice receiving NT siRNA ( n =21) post-injury displayed decreased alternating behaviour to a mean of 48.8%, while mice receiving claudin-5 siRNA ( n =21) post-injury showed a significant increase in alternating behaviour (* P ≤0.05, ANOVA with Tukey's post-test) with a mean of 60.5% alternating behaviour. ( f ) Four individual siRNAs designed to target different regions of the human claudin-5 mRNA were designed and screened using qPCR. All siRNA's displayed efficient suppression (*** P ≤0.0001, ANOVA with Tukey's post-test, n =3 for each group) and claudin-5 siRNA 1 and claudin-5 siRNA 3 were chosen because of their target region homology with all major non-human primates. ( g ) Western blot analysis of claudin-5 levels post-transfection of claudin-5 siRNA 1 and claudin-5 siRNA 3 showed efficient suppression of claudin-5 at the protein level. Full size image TUNEL analysis of mice receiving NT siRNA or claudin-5 siRNA showed a decreased amount of apoptotic/necrotic cells at the penumbra, when claudin-5 was suppressed ( Fig. 8c ). This decrease in cell death was localized to the CA1 region of the hippocampus ( Fig. 8b ) and, in this regard, we sought to use a hippocampal-linked spontaneous alternation behavioural task in the T-maze ( Fig. 8d ) [29] , [30] . Mice were analysed 2 weeks post-injury and were divided into groups of animals receiving NT siRNA or mice receiving claudin-5 siRNA post-injury. Sham (un-injured) animals were used to achieve a baseline experimental readout. Mice receiving claudin-5 siRNA performed significantly better in the T-maze assessment compared with NT siRNA-injected mice ( Fig. 8e ). Identification of optimum siRNA for human use We sought to identify an siRNA with a target region for optimum suppression of human claudin-5 with exact homology between a range of primate species. To this end, we identified four distinct siRNAs with varying suppression efficacies. We then chose two of these siRNAs and analysed the sequence homology of the target region of the messenger RNA in all major non-human primates compared with human ( Supplementary Table S3 ). siRNAs termed 'CLDN5 siRNA 1' and 'CLDN5 siRNA 3' gave highly efficient suppression of claudin-5 in human endothelial cells ( Fig. 8f ), when analysed in cell culture models, and will be used for pre-clinical safety/toxicology studies in non-human primates before human clinical trials of claudin-5 siRNA ( Fig. 8g ). Cerebral oedema associated with TBI is the leading cause of death and disability in children and young adults globally. Added to this, is the malignant brain oedema seen in 10% of ischemic strokes, the greater than 90% mortality associated with hypoxic ischemic injury post-cardiac arrest and the high morbidity and mortality associated with brain cancer and infection. Sadly, the costs associated with its consequences and, often, futile treatments [31] , [32] , [33] , which have remained unchanged in almost a century, put immense economic burden on families and society in general. One of the key mediators of increased ICP is a dramatic shift in water diffusion across the BBB [4] , [34] . While it is well accepted that the BBB is damaged in cases of TBI, the BBB becomes dysfunctional and levels of expression of a range of tight junction proteins are transcriptionally increased or decreased at varying time points post-injury [20] . Moreover, the dramatic neuroinflammatory response, observed in cases of cerebral oedema, causes the upregulation of a range of cytokines that may have the potential to impact on the integrity of the tight junction on the BBB [25] . There is no available animal model of TBI that reflects all of the heterogenous characteristics of a human TBI. Controlled cortical impact is a common technique used for establishing cerebral oedema in rodent models, and the extent of brain swelling that occurs in rodents, following a controlled-cortical impact to the brain, is significant [35] . In this model, brain swelling extends out of the skull due to the presence of a 'burr hole' ( Supplementary Fig. S6 ); however, in the vast majority (up to 90%) of TBI incidents in humans, swelling and oedema are confined to the skull in non-penetrating injuries [36] . We sought to use a focal injury, the mouse cortical cold injury model, which has previously been used extensively to study the dynamic of cerebral oedema formation [37] , [38] , [39] . This model has been shown to cause changes in caveolin-1, occludin and claudin-5 expression within the lesion site at various time points post-injury and highlights the dynamic changes that occur with respect to the BBB post-neuronal injury [20] . Interestingly, the dynamic of BBB dysfunction was observed to differ over time in this model of cerebral oedema. Mice receiving claudin-5 siRNA post-injury showed a marked difference in the pattern of Gd-DTPA extravasation compared with NT siRNA in the penumbra, with contrast still evident 48 h post-injury, indicative of a modulated BBB in this region. Also, in relation to the cytokine profile at the site of injury, we believe that the increased levels of IL-1β and CXCL10 observed may have fundamental protective roles in early stage suppression and prevention of excessive cerebral oedema formation and will warrant significant further study. Our findings show that, using BBB modulation, enhanced exchange of water in the brains of mice with a focal brain injury for a period of between 24 and 72 h in a controlled and reversible sense, provides a positive outcome with respect to lesion size and vascular perfusion (rCBV) at the site of injury. In addition, systemic administration of claudin-5 siRNA has a good safety profile in mice. Indeed, siRNA/ in vivo-jetPEI complexes are currently being used in a Phase I clinical trial and in vivo-jetPEI has already been approved for systemic use by the US Food and Drug Administration ( http://www.polyplus-transfection.com / ). Although there have been many clinical trials for novel treatments of TBI since the mid-1990s, the results have been largely disappointing. [40] Many reasons have been cited for these negative results, yet, a large majority of these trials focussed on the administration of neuroprotective agents to treat the secondary effects of trauma and not on mitigating cerebral oedema itself. Given our observations that the dysfunctional BBB will not allow for the passive diffusion of small molecules at distinct time points post-injury, it is not surprising that these neuroprotective agents had minimal effect owing to their possible inability to diffuse from the blood into the parenchyma and, more importantly, the penumbra. Our observations may have profound consequences for early intervention treatment of cases of TBI and other causes of acute brain injury, and may facilitate significant decreases in cerebral oedema following injury. Indeed, in many cases of TBI and stroke (where initial cytotoxic oedema can lead to vasogenic oedema), there are delayed effects on the brain that may lead to swelling. In addition, the secondary tissue injury processes may be set in motion, some time after the initial insult, and so a longer phase of barrier opening would be of importance. Overall, our findings could have major applications in a range of neurological conditions, where cerebral oedema is the central cause of morbidity and mortality and where uncontrolled brain swelling can be catastrophic in the most extreme cases. Animal experiments and experimental groups All studies carried out in the Smurfit Institute of Genetics in TCD adhere to the principles laid out by the internal ethics committee at TCD, and all relevant national licences were obtained before commencement of all studies. C57/Bl6J were sourced from Jackson Laboratories and bred on-site at the Smurfit Institute of Genetics in Trinity College Dublin (TCD). Cerebral oedema model Briefly, an anaesthetized mouse was mounted on a stereotaxic frame, an incision was made in the scalp, and the skull exposed. A controlled cold-induced brain injury was inflicted using a 4–mm diameter metal rod supercooled with liquid N 2 . The metal rod was placed on the skull using exact stereotaxic co-ordinates (2 mm behind bregma, 2 mm right lateral), and with a 'downward weight' of 100 g, the rod was left in place for 30 s causing focal oedema in the visual and somatosensory cortex extending as deep as CA1 of the hippocampus. Un-injured control mice were surgically prepared in a similar manner, but they were not subjected to injury. Following injury, the scalp was sutured and mice were housed in a recovery chamber at 37 °C. Sham, and injured mice were allowed to recover from anaesthesia, and within 1 h of the injury were injected with NT or claudin-5 siRNA/ in vivo-JetPEI ™. Web-based siRNA design protocols targeting claudin-5 Sequences of the claudin-5 siRNA used in this study were from Dharmacon and were as follows. Sense sequence: 5′-CGUUGGAAAUUCUGGGUCUUU-3′. Antisense sequence: 5′-AGACCCAGAAUUUCCAACGUU-3′. Non-targeting control siRNA-targeting luciferase was used as a non-targeting control sense sequence: CUUACGCUGAGUACGUCGAdTdT. Antisense sequence: UCGAAGUACUCAGCGUAAGdTdT. 2′OMe-modified claudin-5 siRNA was synthesized by Dharmacon and were as follows: sense sequence: 5′-CGUmUGGAAAUUCUGmGGUCUUU-3′. Antisense sequence: 5′-AGACCCAGAAUUUCCAACGUU-3′, where 'm' prefixing a nucleotide indicates 2′OMe modification at this residue. Cell culture and transfection One day before transfection, 1×10 5 mouse bEnd.3. (ATCC) or human umbilical vein endothelial cells were plated in 500 μl of growth medium in a 24–well plate. 20 pmol NT, or claudin-5 siRNAs were transfected per well using Lipofectamine 2000 (Invitrogen) and RNA or protein isolated after 24, 48, 72, 96 h or 1 week. Mouse BMDMs were isolated from WT C57/Bl6 mouse bone marrow. In vivo delivery of siRNA Claudin-5 siRNA (20 μl of 1 μg μl −1 ) was diluted in 100 μl of a 10% glucose solution. The volume was adjusted to 200 μl using RNAse/DNAse free water. Solutions were mixed and briefly centrifuged. In a separate tube, 6.4 μl in vivo-jetPEI ™ (Catalogue no. 201–50) was diluted in 100 μl of a 10% glucose solution. The volume was adjusted to 200 μl, using RNAse/DNAse free water, and solutions were briefly mixed. The 200 μl in vivo-jetPEI ™ solution was then added to the siRNA solution, vortexed and briefly centrifuged. Solutions were then incubated for 15 min, at room temperature, to allow complexes to form. Mice were injected slowly in the tail vein (400 μl final volume per mouse). Analysis of zeta-potential Following complexing of siRNA with in vivo-jetPEI ™, zeta-potential was assessed using a zeta-sizer (Malvern Instruments). Particle size was also determined using the same system. Brain microvasculature fractionation and western analysis Brains were homogenized in 5 ml DMEM and spun at 3,000 r.p.m., for 5 min. The homogenate was dissociated with 0.005% (wt/vol) dispase (grade 1; Roche Diagnostic) at 37 °C, for 2 h. Homogenates were centrifuged at 3,000 r.p.m. for 5 min and pellets were re-suspended in a dextran solution ( M w 70,000; 10% wt/vol; Sigma) and centrifuged at 3,000 r.p.m. at 4 °C for 10 min. Pellets were re-suspended with PBS and centrifuged at 800 g for 5 min. The final pellet was re-suspended in protein lysis buffer (62.5 mM Tris, 2% SDS, 10 mM Dithiothreitol, 10 μl protease inhibitor cocktail/100 ml (Sigma Aldrich), centrifuged at 12,000 r.p.m. for 20 min at 4 °C and supernatant removed for claudin-5 analysis. Antibodies for western blot were as follows: polyclonal rabbit anti-claudin-5 (Zymed Laboratories, San Francisco, California, USA) (1:500), polyclonal rabbit anti-β-actin (Abcam, Cambridge, UK) (1:1,000). Indirect immunostaining of brain cryosections Briefly, rabbit anti-claudin-5 (Zymed), was incubated on sections overnight at 4 °C. Secondary rabbit IgG-Cy3, (Jackson-Immuno-research, Europe) antibodies were incubated with the sections at 37 °C for 2 h followed by 3 washes with PBS. All sections were counterstained with DAPI for 30 s at a dilution of 1:5,000 of a stock 1 mg ml −1 solution. Post-mortem and histopathological evaluations Post-mortem examinations were undertaken immediately following euthanasia. To assess multiple organs for toxicity, samples of the brain, liver, lung, heart, kidneys, spleen, pancreas, thymus, oesophagus and adrenal glands were immediately fixed in formalin. Following fixation tissues were paraffin-embedded, sectioned at 5 μm and stained with haematoxylin & eosin. Similar processing and staining procedures were used to evaluate the brain histopathological changes in the TBI model. Magnetic resonance imaging Following administration of TBI and subsequent siRNA injection, BBB integrity was assessed in vivo via MRI, using a dedicated small rodent 7 T MRI system located at TCD ( http://www.tcd.ie/Neuroscience/infrastructure/neuroimaging/index.php#7tesla ). To visualize brain damage and lesion volumes, high-resolution images were acquired using Rapid Acquisition with Relaxation Enhancement (RARE) two-dimensional sequence with a RARE factor of 8 and an echo time resulting in an effective time of 42.2 ms (with a flip angle of 180°). With an acquisition matrix of 128×128 and a field of view of 1.8 cm 2 ×1.8 cm 2 , the pixel resolution was 0.141 mm per pixel. In the coronal plane, 15 slices, each measuring 0.25 mm in thickness were acquired. Repetition time was 7,274.2 ms, and 4 averages were used for a total measuring time of 7 min 45 s. Compromises of the BBB were then visualized in high-resolution T1 weighted MR images (resolution, 0.156 mm×0.156 mm×5 mm; field of view: 20 mm×20 mm×17.9 mm 3 ; matrix; 128×128×30; TR/TE: 500/2.7 ms; flip angle: 30° number of averages: 3; acquisition time: 2 min, 24 s; repetitions: 12) following administration of 100 μl of a 1 in 3 dilution of Gd-DTPA (Gadolinium diethylene-triamine penta-acetic acid), administered via the tail vein. A more quantitative assessment of BBB compromise was also made using dynamic contrast-enhanced MRI, in which the passage of Gd-DTPA from the vasculature into the tissue was monitored over a period of 20 min post-injection (referred to above as 'bolus chase analysis'). The ASL sequence consisted of the preparation interval that contained the inversion pulse to magnetically label inflowing arterial blood water in the neck, followed by a variable post-labelling delay and then snapshot fast low angle shot acquisition in the brain. Parameters used were as follows: slice thickness=2 mm, fast low angle shot TR=6.938 ms, echo time TE=2.63 ms, RF flip angle=30° FOV=3.0×3.0 cm, image matrix=128×64, receiver bandwidth=100 kHz. Values for MTT, CTT and rCBV were quantified using a non-compartmental model of cerebral perfusion [23] , [24] . Real-time PCR TBI regions were excised from brain tissue and RNA isolated using the RNeasy Mini Kit (Qiagen). Genomic DNA was eliminated by the addition of DNase as per the manufacturer's instructions. RNA was quantified using the Quantitect SYBR Green Kit (Qiagen-Xeragon) in a 7300 Real-Time PCR System under the following reaction conditions: 50 °C×20 min, 95 °C×15 min, [95 °C×15 s, 60 °C×1 min]×37, 95 °C×15 s, 60 °C×1 min, 95 °C×15 s, 60 °C×15 s. Primers were supplied by Sigma-Aldrich and were as follows: NGF left: 5′-CCGCAGTGAGGTGCATAG-3′ and right: 5′-GCTTCAGGGACAGAGTCTCC-3′; IL-1–left: 5′-TCAGGCAGGCAGTATCACTC-3′ and right: 5′-AGGATGGGCTCTTCTTCAAA-3′; ICAM-1 left: 5′-CCATCACCGTGTATTCGTTT-3′ and right: 5′-GAGGTCCTTGCCTACTTGCT-3′; CINC-1 left: 5′-CCGAAGTCATAGCCACACTC-3′ and right: 5′-GTGCCATCAGAGCAGTCTGT-3′; RANTES left: 5′-TCTTGCAGTCGTGTTTGTCA-3′ and right: 5′-GGGTCAGAATCAAGAAACCC-3′. Transcript levels were standardized using β-actin, and calculated using the ΔΔCT method. RNA isolated from siRNA-transfected human umbilical vein endothelial cells cells was quantified, using the same reaction conditions with the following primers, Claudin-5 left: 5′-CTGGACCACAACATCGTGA-3′ and right: 5′-CACCGAGTCGTACACTTTGC-3′ and β-actin left: 5′-GGGAAATCGTGCGTGACAT-3′ and right: 5′-GTGATGACCTGGCCGTCAG-3′. Transcriptional changes were also measured in a StepOne Plus machine (Applied Biosystems), using Taqman Gene Expression Assays (Applied Biosystems) with the following IDs: IL10 (Mm00439614_m1), CXCL10 (Mm00445235_m1), TGF-β1 (Mm00441726_m1), TNF-a (Mm99999068_m1), VCAM-1 (Mm01320970_m1), GDNF (Mm00599849_m1), BDNF (Mm04230607_s1) IFN-a (Mm00833961_s1). All target genes used a FAM reporter. Reaction conditions were as follows: 50 °C×2 min, 95 °C×20 s, [95 °C×1 s, 60 °C×20 s]×40. Transcript levels were standardized using β-actin with a VIC reporter in the same well, and calculated using the ΔΔCT method. Neurological severity score assessments A measure of neurological severity was obtained using ten tests for markers of motor and cognitive function, as previously described [28] . The tests were performed by an individual blinded to the experimental treatment and were as follows: exit a circle with a diameter of 30 cm within 3 min; ability to use all 4 limbs; initiative and ability to walk straight; startle reflex; seeking behaviour; ability to balance on a beam 7 mm wide for 10 s; cross a 30 cm beam of width 3 cm in 3 min; same test, beam narrowed to 2 cm; same test, beam narrowed to 1 cm; ability to perch on a round beam of width 5 mm. TUNEL analysis To detect cell death, fixed brain sections were incubated with staining mix (in situ Cell Death Detection kit, TMR red, Roche), according to manufacturer's instructions, for 1 h at 37 °C in the dark, followed by 2 washes in PBS for 5 min each in the dark. Sections were visualized at room temperature using a fluorescent microscope (Zeiss Axioplan 2, Oberkochen, Germany) with integrated software. Hippocampal-linked spontaneous alternation task In our experiment, testing began on recovery day 14 to minimize motor impairments produced by TBI and performed by a blinded observer. Each mouse is placed in the stem arm (start area) and then released to choose one of the goal arms. Once the mouse enters the chosen arm, it is confined there for 30 s by closing the goal arm door. The animal is then placed back at the start area for 15 s (stem arm door closed) and released (stem arm door opened) to again choose one of the two goal arms. If the second choice is different from the first choice, then the mouse is scored as 'alternating' for the trial. Mice are tested for 8 days with 3 trials per day. The per cent alternation over the duration of testing was calculated for each animal. Experiment was done in constant dim light at 22±2 °C (refs 40 , 41 ). Statistical analyses Statistical analysis was performed using Student's t -test, with significance represented by a P -value of ≤0.05. For multiple comparisons, ANOVA was used with a Tukey-Kramer post test and significance represented by a P -value of ≤0.05. For ASL analysis, ANOVA followed by a Bonferroni post test for multiple comparisons was used with P ≤0.05 representing significance. How to cite this article: Campbell, M. et al . Targeted suppression of claudin-5 decreases cerebral oedema and improves cognitive outcome following traumatic brain injury. Nat. Commun. 3:849 doi: 10.1038/ncomms1852 (2012).